Dynamically stabilized magnetic skyrmions Magnetic skyrmions are topologically non-trivial spin textures that manifest themselves as quasiparticles in ferromagnetic thin films or noncentrosymmetric bulk materials. So far attention has focused on skyrmions stabilized either by the Dzyaloshinskii–Moriya interaction (DMI) or by dipolar interaction, where in the latter case the excitations are known as bubble skyrmions. Here we demonstrate the existence of a dynamically stabilized skyrmion, which exists even when dipolar interactions and DMI are absent. We establish how such dynamic skyrmions can be nucleated, sustained and manipulated in an effectively lossless medium under a nanocontact. As quasiparticles, they can be transported between two nanocontacts in a nanowire, even in complete absence of DMI. Conversely, in the presence of DMI, we observe that the dynamical skyrmion experiences strong breathing. All of this points towards a wide range of skyrmion manipulation, which can be studied in a much wider class of materials than considered so far. Magnetic skyrmions are topologically non-trivial whirls in the magnetization field which, unlike vortices, leave the ferromagnetic state intact far away from their core. The corresponding two-dimensional magnetization field with a configuration space of a two-sphere is smooth and wraps around the unit sphere an integer number of times thus endowing a skyrmion with topological stability. These remarkable objects [1] , [2] , [3] , [4] , [5] , [6] , [7] , [8] , [9] were initially observed as flux lattices in ferromagnets without inversion symmetry such as MnSi and Fe 0.5 Co 0.5 Si (refs 10 , 11 ) and later also in thin films of similar materials [11] , [12] . In these B20-type materials, skyrmions are inherently chiral objects that are stabilized by the parity breaking Dzyaloshinskii–Moriya interaction (DMI) that may exist in noncentrosymmetric ferromagnets. In some instances, even control of whole skyrmion lattices has been achieved [13] . However, to unleash their extraordinary potential as next-generation information carriers, control of individual skyrmions has to be achieved. Isolated skyrmions have been proposed to exist in ultra-thin magnetic nanowires where asymmetric interfaces provide the necessary DMI [14] , [15] , [16] . These hedgehog skyrmions (cf. Fig. 1 ) can be nucleated and transported along a sample as shown numerically [14] . The controlled creation and deletion of isolated DMI stabilized skyrmions was recently demonstrated experimentally in one monolayer of Fe grown on Ir(111) with the aid of spin-polarized tunnelling microscopy [17] . 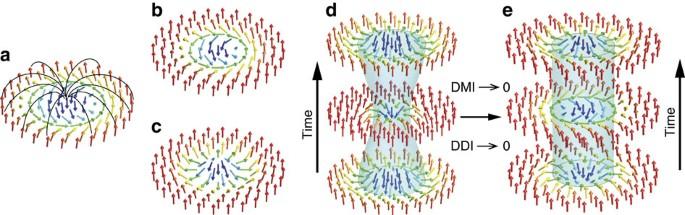Figure 1: Different skyrmion stabilization mechanisms. Panels (a–e) show skyrmions with skyrmion number. (a) A bubble skyrmion stabilized by dipolar interactions which may exist as a left- or right-handed version. Its size typically exceeds that of skyrmions stabilized by DMI. (b,c) DMI stabilized skyrmions: (b) A chiral skyrmion as favoured in B20-type materials such as MnSi. (c) A hedgehog skyrmion as favoured by interfacial DMI. Note that in both cases the domain-wall chirality when passing through the skyrmion centre is fixed by the DMI and not degenerate as ina. (d) Dynamically stabilized magnetic skyrmion which requires neither dipolar interactions nor DMI and which exhibits precession around the (vertical) easy-axis anisotropy. During precession, the skyrmion number is strictly conserved and the skyrmion sweeps across all possible chiral and hedgehog configurations. In the presence of either dipolar interactions, DMI, or an Oersted (Oe) field, the skyrmion diameter varies periodically in time (breathing). (e) For vanishing dipolar interactions (DDI), DMI and Oe fields, and in absence of damping, the skyrmion precesses uniformly and breathing disappears. Note that paneleonly shows half a period of the precessional motion to emphasize that both chiral and hedgehog configurations are being covered in the DS states. Figure 1: Different skyrmion stabilization mechanisms. Panels ( a – e ) show skyrmions with skyrmion number . ( a ) A bubble skyrmion stabilized by dipolar interactions which may exist as a left- or right-handed version. Its size typically exceeds that of skyrmions stabilized by DMI. ( b , c ) DMI stabilized skyrmions: ( b ) A chiral skyrmion as favoured in B20-type materials such as MnSi. ( c ) A hedgehog skyrmion as favoured by interfacial DMI. Note that in both cases the domain-wall chirality when passing through the skyrmion centre is fixed by the DMI and not degenerate as in a . ( d ) Dynamically stabilized magnetic skyrmion which requires neither dipolar interactions nor DMI and which exhibits precession around the (vertical) easy-axis anisotropy. During precession, the skyrmion number is strictly conserved and the skyrmion sweeps across all possible chiral and hedgehog configurations. In the presence of either dipolar interactions, DMI, or an Oersted (Oe) field, the skyrmion diameter varies periodically in time (breathing). ( e ) For vanishing dipolar interactions (DDI), DMI and Oe fields, and in absence of damping, the skyrmion precesses uniformly and breathing disappears. Note that panel e only shows half a period of the precessional motion to emphasize that both chiral and hedgehog configurations are being covered in the DS states. Full size image In magnetic films there exists another class of localized objects often referred to as bubbles which may share the topology of chiral skyrmions. Being stabilized entirely by the parity preserving dipolar interactions, such bubble skyrmions [18] , [19] can exist with either handedness but are typically larger than their DMI-induced counterparts. In nanodisks they have recently been observed to exhibit a surprisingly large mass [20] . In addition to these two classes of objects, DMI stabilized skyrmions and bubble skyrmions, we now demonstrate the existence of a third one, a dynamically stabilized magnetic skyrmion that shares its topology with its well-known siblings, but which derives its existence from precessional dynamics only. It exists even when dipolar interactions and DMI are absent, and it is dynamically stabilized by the coherent internal precession of its moments around the anisotropy axis while its diameter is in general oscillating with time, an effect known as breathing. Unlike DMI stabilized skyrmions and bubbles that have quasistatic character and correspond to a metastable state of the micromagnetic energy, such a dynamical skyrmion (DS) constitutes a quasiparticle that can be nucleated and sustained indefinitely under a nanocontact (NC) with spin transfer torque, while it has a finite lifetime outside the lossless environment of the NC. Remarkably, however, it can be transported coherently through the energetically unfavourable environment of a dissipative medium between well separated NCs even when DMI is absent. Since the DS always recovers its initial state on reaching a NC, coherent propagation over large distances involving several NCs is possible. In the presence of DMI, the dynamical magnetic skyrmion exhibits strong breathing which opens the avenue for skyrmion-based memory and microwave applications. We develop an analytic theory to demonstrate the generic nature of the DS, which explicitly demonstrates that its sustenance does not depend on the magnitude of DMI and is possible even in its absence. The DS is the topologically non-trivial counterpart of the precessional magnetic droplet [21] , whose existence was recently experimentally demonstrated [22] in NC-spin torque oscillators. While originally considered a theoretical curiosity, only stable in films with strong perpendicular anisotropy with zero spin wave damping [23] , [24] , the advent of spin transfer torque [25] , [26] made it possible to locally create an effectively lossless spin wave medium [27] , [28] with the required material properties for droplet nucleation and manipulation [21] , [29] . DSs as a generic solution We start by demonstrating that the DS can be nucleated in a NC and exists as a generic solution even in absence of DMI and dipolar interaction. These latter interactions are necessary for the stabilization of chiral DMI skyrmions or bubble-type skyrmions. As a starting point, we micromagnetically [30] model a NC-spin torque oscillator in zero applied field with an ultra-thin Co layer with strong perpendicular anisotropy, without any DMI, and neglecting dipolar interactions (for micromagnetic details, see Methods section). As expected, we nucleate an ordinary magnetic droplet above a critical current given by the Slonczewski instability to auto-oscillations [21] . The droplet is characterized by a reversed core, with all spins precessing in phase, and is topologically trivial as it can be continuously transformed into the uniform ferromagnetic state. On increasing the current density we find that there exists a second, higher, threshold current above which, instead of a droplet, we excite a precessing object with a non-zero skyrmion number ( n =− m ·(∂ x m × ∂ y m ) being the topological density [19] , [31] and m the magnetization unit vector). 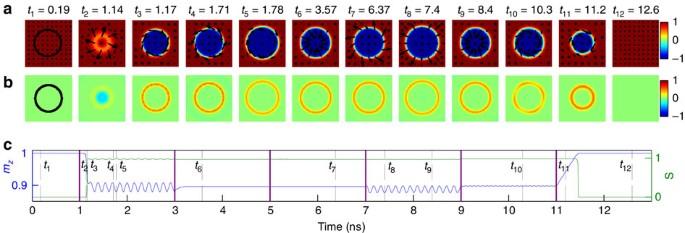Figure 2: Nucleation and tuning of a DS. Micromagnetic simulation of a NC-spin torque oscillator with radius 40 nm and atJ=6 × 108A cm−2showing the nucleation of a DS without DMI and dipolar interactions from an initial ferromagnetic (FM) state and the subsequent tuning of the DS by spin transfer torque,α, DMI, and dipolar interaction. (a) Top view of the spin structure at different times of the simulation; the black circle indicates the NC; The blue and red colour of the colour bar represent the downward (mz=−1) and upward (mz=+1) orientations of the magnetizations, respectively. (b) top view of the topological density at the same times as ina; (c) Time trace of the out-of-planemzcomponent averaged over the simulation area and time trace of the skyrmion number; dashed vertical lines correspond to the snapshots above. For 0<t<1 ns, the system undergoes an initial relaxation from FM state. For 1 ns<t<3 ns, a DS is nucleated under finite spin transfer torque assisted by the corresponding Oe field without DMI. For 3 ns<t<5 ns, the Oe field is artificially turned off and the breathing disappears. For 5 ns<t<7 ns, both current and damping are turned off. For 7 ns<t<9 ns, a moderate DMI is added and the breathing resumes. For 9 ns<t<11 ns, we only turn on dipolar interactions (both Oe field and DMI are off) and minor breathing is again observed. For 11 ns<t<13 ns, the DS will dissipate into a uniform ferromagnetic state if only damping is turned on without spin torque. Figure 2 presents the simulation results, with Fig. 2a displaying snapshots of the top view of the free-layer magnetization, Fig. 2b the corresponding topological density, and Fig. 2c the time trace of the average out-of-plane magnetization component m z and the corresponding skyrmion number (see also Supplementary Movie 1 ). After an initial relaxation, a current density of J =6 × 10 8 A cm −2 is switched on. The system first forms a doughnut structure at times t 2 and t 3 , due to the Oersted (Oe) field and at time t 4 eventually forms a dynamically precessing object, characterized by a fully reversed core, spins precessing along its perimeter, and . This state retains the dynamical precessing character of the droplet, while having the topology of a skyrmion, and hence constitutes a DS. Contrary to the droplet, where all spins precess in phase, the spins along the perimeter of the DS undergo a 2 π rotation (cf. Fig. 1c ), leading to continuous transformations between hedgehog and vortex-like spin textures [32] , while always retaining a skyrmion number of 1. The spatially averaged in-plane magnetisation is hence constant in time. However, because of the large static Oe field, the DS experiences a time-varying Zeeman energy and as a consequence exhibits breathing at exactly the precession frequency; if we artificially turn off the Oe field ( t =3 ns) the breathing disappears. The breathing causes a strong variation in m z that allows us to unambiguously determine the precession frequency. This behaviour is reminiscent of the breathing observed in quasi-one-dimensional magnetic soliton-antisoliton pairs [33] and which also exists in one-dimensional soliton–soliton breathers [34] . Figure 2: Nucleation and tuning of a DS. Micromagnetic simulation of a NC-spin torque oscillator with radius 40 nm and at J =6 × 10 8 A cm −2 showing the nucleation of a DS without DMI and dipolar interactions from an initial ferromagnetic (FM) state and the subsequent tuning of the DS by spin transfer torque, α , DMI, and dipolar interaction. ( a ) Top view of the spin structure at different times of the simulation; the black circle indicates the NC; The blue and red colour of the colour bar represent the downward ( m z =−1) and upward ( m z =+1) orientations of the magnetizations, respectively. ( b ) top view of the topological density at the same times as in a ; ( c ) Time trace of the out-of-plane m z component averaged over the simulation area and time trace of the skyrmion number; dashed vertical lines correspond to the snapshots above. For 0< t <1 ns, the system undergoes an initial relaxation from FM state. For 1 ns< t <3 ns, a DS is nucleated under finite spin transfer torque assisted by the corresponding Oe field without DMI. For 3 ns< t <5 ns, the Oe field is artificially turned off and the breathing disappears. For 5 ns< t <7 ns, both current and damping are turned off. For 7 ns< t <9 ns, a moderate DMI is added and the breathing resumes. For 9 ns< t <11 ns, we only turn on dipolar interactions (both Oe field and DMI are off) and minor breathing is again observed. For 11 ns< t <13 ns, the DS will dissipate into a uniform ferromagnetic state if only damping is turned on without spin torque. Full size image If we simultaneously turn off both current and damping ( t =5 ns), the DS remains in a stationary precessing state due to the absence of dissipation. Although this corresponds to an idealized case, it indicates that the DS is a generic conservative soliton solution for a DMI-free film with perpendicular magnetic anisotropy in zero field. If we add a moderate DMI of 0.2 mJ m −2 ( t =7 ns) m z again varies in time and breathing resumes. If instead of DMI and Oe field we only turn on dipolar interactions ( t =9 ns), minor breathing is again observed, but this time at twice the precession frequency [24] . Finally, if only damping is turned on ( t =11 ns), the DS transforms into a uniform ferromagnetic state, accompanied with an emission of spin waves as shown in the Supplementary Movie 1 . As the skyrmion number changes in this process, the skyrmion annhiliation occurs via a Bloch point (cf. ref. 35 ), a process that is discussed in detail in Supplementary Fig. 1 . This again clearly demonstrates that the DS is not an excited state or an eigenmode of a static skyrmion, but a fundamental solution in the form of a precessing skyrmion without the necessity of DMI or dipolar interactions. As seen in Fig. 3a,b the NC size and the strength of the perpendicular magnetic anisotropy ( K u ) controls the overall frequency and radius of the DS, which can then be further actively tuned by the drive current: higher current increases the DS radius and red shifts its frequency. It is also possible to reduce the drive current well below the nucleation current without losing the DS. Similar to the droplet, the sustaining current of the DS can hence be much smaller than its nucleation current, resulting in a very large hysteresis in current. 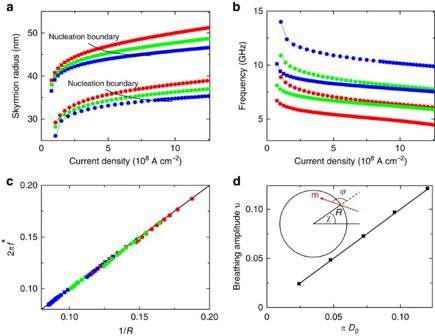Figure 3: Linear scaling law of a DS. (a) DS radius versus current density for two NC sizes and three different strengths of the perpendicular magnetic anisotropy; (b) DS frequency as function of current density; (c) Linear scaling law between the DS frequency and inverse radius, for currents at threshold and below, in excellent agreement with the analytical prediction. For panels (a–c): red square corresponds to NC radius of 40 nm andKu=0.5 MJ m−3; green square corresponds to NC radius of 40 nm andKu=0.7 MJ m−3; blue square corresponds to NC radius of 40 nm andKu=1 MJ m−3; red dot corresponds to NC radius of 30 nm andKu=0.5 MJ m−3; green dot corresponds to NC radius of 30 nm andKu=0.7 MJ m−3; blue dot corresponds to NC radius of 30 nm andKu=1 MJ m−3. (d) The DMI-induced breathing amplitudeν=(Rmax−Rmin)/(Rmax+Rmin) as a function ofD0, in which the simulation results are again in excellent agreement with the theory. The filled square represents the micromagnetic simulation results and the solid line represents the theory. The inset shows coordinates used in the theory: χ is the (real space) polar angle,Ris the skyrmion radius, and φ the azimuthal angle of the magnetizationmrelative to the radial direction. For main panelsa–c, the Gilbert damping coefficientα=0.3, with no DMI but with Oe field. Figure 3: Linear scaling law of a DS. ( a ) DS radius versus current density for two NC sizes and three different strengths of the perpendicular magnetic anisotropy; ( b ) DS frequency as function of current density; ( c ) Linear scaling law between the DS frequency and inverse radius, for currents at threshold and below, in excellent agreement with the analytical prediction. For panels ( a – c ): red square corresponds to NC radius of 40 nm and K u =0.5 MJ m −3 ; green square corresponds to NC radius of 40 nm and K u =0.7 MJ m −3 ; blue square corresponds to NC radius of 40 nm and K u =1 MJ m −3 ; red dot corresponds to NC radius of 30 nm and K u =0.5 MJ m −3 ; green dot corresponds to NC radius of 30 nm and K u =0.7 MJ m −3 ; blue dot corresponds to NC radius of 30 nm and K u =1 MJ m −3 . ( d ) The DMI-induced breathing amplitude ν =( R max − R min )/( R max + R min ) as a function of D 0 , in which the simulation results are again in excellent agreement with the theory. The filled square represents the micromagnetic simulation results and the solid line represents the theory. The inset shows coordinates used in the theory: χ is the (real space) polar angle, R is the skyrmion radius, and φ the azimuthal angle of the magnetization m relative to the radial direction. For main panels a – c , the Gilbert damping coefficient α =0.3, with no DMI but with Oe field. Full size image These numerical results can be understood in terms of an effective analytical model. The cylindrical symmetry of the DS lends itself to a description with the skyrmion radius R ( t ) and the relative azimuthal angle as dynamical variables (for details see inset of Fig. 3d ) while assuming that R is considerably larger than the static domain-wall width which is satisfied in our simulations. On the basis of a two-dimensional energy density that contains exchange, anisotropy, DMI, dipolar interactions and an Oe field, (cf., for example, ref. 36 ), the Landau–Lifshitz–Gilbert–Slonczewski equation leads to the following effective equations of motion (cf. Supplementary Note 1 ) The dot indicates a derivative with respect to time which is measured in units of the inverse anisotropy frequency M s /2 γK u . The skyrmion radius R is defined as the radius of the circle where m z =0 and is measured in units of the domain-wall width , where A is the micromagnetic exchange stiffness. is a function containing contributions from DMI, Oe fields and dipolar interactions, α is the damping constant, denotes the dimensionless spin-torque amplitude which is defined in the Methods section, and denotes the Heaviside step function smoothed over a length δ 0 , and a c is the radius of the NC measured in units of δ 0 (for details see Supplementary Note 1 ). Equations (1 hold under the assumption that R >1. The first order differential equations capture the essence of the skyrmion dynamics observed in numerical simulations shown in Fig. 2 . In the idealized case of an undamped and undriven system, , the instantaneous skyrmion radius and precession frequency obey the simple relation, where is measured in units of the anisotropy frequency. As illustrated in Fig. 3c , our micromagnetic simulations follow this relation very closely without any adjustable parameters and even in presence of nonvanishing currents and finite damping, if the time average is taken over one period. Considering the fact that we map a micromagnetic system with many degrees of freedom onto an effective system with only two dynamical variables, such quantitative agreement is quite remarkable. In the idealized case without DMI, Oe fields and dipolar interactions, m z is conserved, and F =0. In this case, both R and are constant in time, and a skyrmion with constant radius is stabilized by uniform precession around the easy axis, which satisfies at all times. Such a precessional DS can exist even in the absence of DMI, which is also observed in the full micromagnetic simulations (cf. Fig. 2a–c in the interval 5 ns≤ t <7 ns). Similar behaviour persists in the presence of damping and compensating spin torque as is seen from the interval 3 ns≤ t <5 ns. In this case, equations (1, 2) can be reduced to with solutions asymptotically converging to a time independent radius . For , the dynamics yields an ever shrinking skyrmion which eventually disappears due to lattice discreteness effects (cf. Supplemenary Note 1 ). This latter effect is seen in the simulations after t =11 ns. If in turn one of these interactions is nonzero, then F ≠0, m z is no longer conserved, and the time dependence of the precession frequency is obtained from ( Supplementary Note 2 ). In case of vanishing Oe fields, this equation is R -independent and can readily be integrated. The solutions exhibit nonuniform precession and by virtue of equation (3), breathing of the skyrmion. Such breathing is indeed seen in the interval 7 ns≤ t <11 ns of Fig. 2a–c (also refer to Supplementary Fig. 2 ). A breathing skyrmion oscillates between the maximum radius (denoted by R max ) and the minimum radius (denoted by R min ) with corresponding relative azimuthal angles and , respectively, which are in turn determined by the zeroes of . If only DMI contributes then the reversal occurs at and ( t 9 , t 10 in Fig. 2 ). Thus at the largest extension, the skyrmion is in a hedgehog configuration favoured by interfacial DMI. For Oe field h Oe <0 (that is, current flowing downwards as in the simulations) we have and , and thus at the largest radius, the skyrmion is in the energetically favoured tangential configuration oriented in a right handed fashion around the current ( t 5 , t 6 in Fig. 2 ). In these cases, breathing and precession frequency coincide. Finally, if only dipolar interactions contribute, then both time reversal and parity are unbroken and a skyrmion with maximal radius is reached at two values , while . As a consequence, the radial oscillation frequency is twice the azimuthal frequency, which is indeed observed in the simulations in the interval 9 ns< t ≤11 ns. In the case of DMI only, we also can easily compute the breathing amplitude ν on time integration of equation (1) over a half period. This yields ν =( R max − R min )/( R max + R min )= πD 0 with , where D is the DMI constant. This relation is followed strikingly well in the presence of both current and damping as shown in the inset of Fig. 3d . Interestingly, the critical current density for DS nucleation can be reduced dramatically (more than one order of magnitude) by using a smaller damping α , smaller K u , and larger NC size, in accordance with the results of ref. 14 , (see also Supplementary Note 2 and Supplementary Fig. 3 ). Under these conditions, it becomes possible to nucleate a DS with relatively small current density in experiments. Furthermore, we confirmed that the above results and conclusions using a damping of α =0.3 remain qualitatively the same if a much smaller damping of α =0.05 is used (see Supplementary Fig. 4 ). Can the DS exist as a quasiparticle outside the NC? To address this question, we investigated the creation and subsequent release of a DS from a NC and its coherent center of mass motion through a nanowire without DMI but with damping. Thereby the DS continues to exhibit coherent precession, and as shown in Fig. 4 , it is moving along a linear trajectory under the influence of an in-plane current, while its diameter continuously decreases for a damping value of α =0.05 in a DMI-free material. After a distance of 150 nm, the DS is captured by a second NC which restores the skyrmion to its initial size. For the skyrmion transport with increased damping, α =0.08, we refer to the Supplementary Fig. 5 . Since the skyrmion is restored in the second NC, an array of NCs can be used to transport the DS over arbitrarily large distances in a DMI-free material. Supplementary Fig. 6 shows an example for the coherent transport across 400 nm involving four NCs. As the motion presented in Fig. 4 does not require DMI, our proposal opens up an avenue for the investigation of skyrmion dynamics in materials without or with much smaller DMI than that required for the formation of quasistatic chiral skyrmions investigated elsewhere. 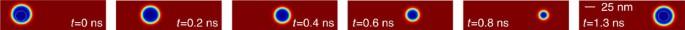Figure 4: Current-induced motion of a DS in a nanowire without DMI. A DS can be transported coherently between NCs along a nanowire without DMI, illustrating its quasiparticle nature. Initially, the skyrmion is nucleated and pinned at the left NC with a diameter of 25 nm. After switching off the spin transfer torque, the DS is released, continues to precess, and is transported coherently by an in-plane current to a second NC at a distance of 150 nm where it is trapped again and restored to its original size. Here the in-plane current density is 1.8 × 108A cm−2and the damping constant is set toα=0.05 with sample dimensions of 250 nm × 75 nm × 1 nm. Hereβ=αis chosen but very similar results are obtained forβ≤αsimilar to the case of DMI stabilized skyrmions14. The white circles indicate the NCs. The red and blue colour indicate up and down magnetization, respectively. Figure 4: Current-induced motion of a DS in a nanowire without DMI. A DS can be transported coherently between NCs along a nanowire without DMI, illustrating its quasiparticle nature. Initially, the skyrmion is nucleated and pinned at the left NC with a diameter of 25 nm. After switching off the spin transfer torque, the DS is released, continues to precess, and is transported coherently by an in-plane current to a second NC at a distance of 150 nm where it is trapped again and restored to its original size. Here the in-plane current density is 1.8 × 10 8 A cm −2 and the damping constant is set to α =0.05 with sample dimensions of 250 nm × 75 nm × 1 nm. Here β = α is chosen but very similar results are obtained for β ≤ α similar to the case of DMI stabilized skyrmions [14] . The white circles indicate the NCs. The red and blue colour indicate up and down magnetization, respectively. Full size image DSs in the presence of large DMI After having convinced ourselves that a dynamic skyrmion is a generic solution that exists even without DMI, we now turn to the interesting case where the DS is nucleated and sustained in a material with large DMI. In this case, the DS exhibits very large breathing which is particularly important for applications. As such systems are known to support also static skyrmions [14] , this regime allows the study of interactions and mutual transformations of droplets, DSs and quasistatic skyrmions into each other. 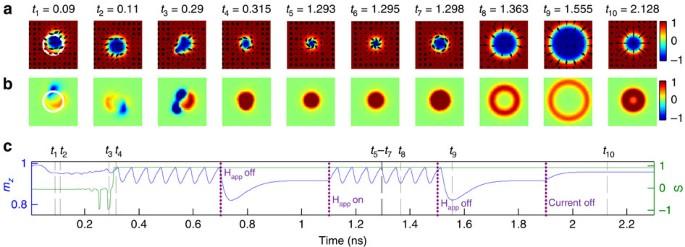Figure 5: Nucleation and field toggling of a DS in presence of DMI. Panels (a–c) show, respectively: the top view of the spin structure at selected simulation times where the white circle indicates the NC of 15 nm radius; the topological density at the same times where the colour-scale is normalized; the time trace of the out-of-plane magnetization componentmzaveraged over the simulation area; and time trace of the skyrmion number (green). Panels (a–c) show droplet nucleation atJ=8.3 × 108A cm−2andμ0Ha=0.3 T, which remains stable for several periods until aboutt=0.2 ns when it becomes increasingly susceptible to anti-skyrmion perturbation. These perturbations eventually (t=0.3 ns) give way to the formation of a DS with. When the applied field is turned off att=0.7 ns, the DS rapidly dissipatively shrinks into a static DMI stabilized skyrmion. If the field is again turned on, the skyrmion can be transformed into a DS in a reversible manner. Finally, if both the field and the current are turned off, the static skyrmion contracts to its equilibrium size given by the material parameters. Figure 5a–c shows the rapid nucleation of a magnetic droplet soliton exhibiting its typical characteristics of precessing spins along its perimeter. Because of the large DMI ( D =3 mJ m −2 ), the spin structure is substantially perturbed ( t 1 and t 2 ) compared with the situation where DMI is absent. At times t 1 and t 2 , regions of weak non-zero topological density are found to rotate around the droplet perimeter. While the droplet is stable for a number of periods the topological perturbations continue to grow in amplitude and almost drive the formation of an anti-skyrmion ( at t 3 ) just before the system switches into a stable state at t 4 . The transition mechanism occurs through a Bloch point pair or a single Bloch point on the surface (cf. Supplementary Note 3 and Supplementary Figs 7 and 8 for details). Figure 5: Nucleation and field toggling of a DS in presence of DMI. Panels ( a – c ) show, respectively: the top view of the spin structure at selected simulation times where the white circle indicates the NC of 15 nm radius; the topological density at the same times where the colour-scale is normalized; the time trace of the out-of-plane magnetization component m z averaged over the simulation area; and time trace of the skyrmion number (green). Panels ( a – c ) show droplet nucleation at J =8.3 × 10 8 A cm −2 and μ 0 H a =0.3 T, which remains stable for several periods until about t =0.2 ns when it becomes increasingly susceptible to anti-skyrmion perturbation . These perturbations eventually ( t =0.3 ns) give way to the formation of a DS with . When the applied field is turned off at t =0.7 ns, the DS rapidly dissipatively shrinks into a static DMI stabilized skyrmion. If the field is again turned on, the skyrmion can be transformed into a DS in a reversible manner. Finally, if both the field and the current are turned off, the static skyrmion contracts to its equilibrium size given by the material parameters. Full size image If the applied field along + z is turned off, the DS relaxes into a static hedgehog skyrmion; if the applied field is again turned on, the DS reforms as the precession restarts. The transition from a DS to a static skyrmion is hence entirely reversible, which is a natural consequence of their identical topology. Finally, if both field and current are turned off, a smaller static hedgehog skyrmion remains with its size given by the DMI and material parameters of the simulation. From the spin transfer torque provided by a non-zero current density, one can controllably tune the size of the static skyrmion, where a positive current density increases its size and a negative current density decreases it. The DS can also be nucleated by controlling only the drive current density. 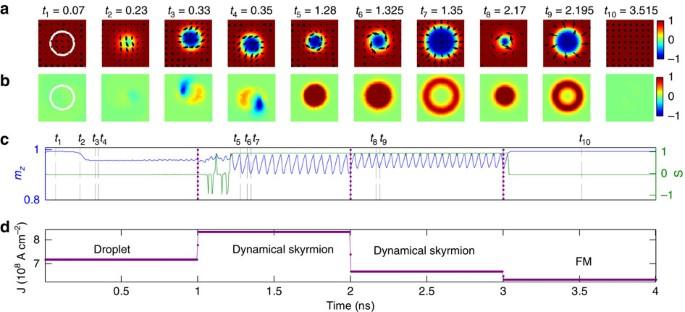Figure 6: Nucleation and current toggling of a DS in presence of DMI. Panels (a–c) show a DS nucleation as a function of current and fixed field, where the white circle indicates the NC of 15 nm radius. For 0 ns<t<1 ns, a magnetic droplet is nucleated whenJ=7.2 × 108A cm−2. For 1 ns<t<2 ns, a DS forms when current density is increased to 8.3 × 108A cm−2. For 2 ns<t<3 ns, a DS remains stable even when the current density is decreased to 6.7 × 108A cm−2, well below the threshold nucleation current density. For 3 ns<t<4 ns, the DS collapses into a uniform ferromagnetic state when the current density is further decreased to 6.3 × 108A cm−2. The current density is varied as follows:J=7.2 × 108A cm−2for 0<t<1 ns, 8.3 × 108A cm−2for 1 ns<t<2 ns, 6.7 × 108A cm−2for 2 ns<t<3 ns, and 6.3 × 108A cm−2for 3 ns<t<4 ns. Panel (d) schematically shows the current pulses applied during the simulation. Figure 6a–d shows a micromagnetic simulation of the same NC-spin torque oscillator in a constant applied field of 0.3 T, which favours a uniform ferromagnetic state. After a period of weak ferromagnetic resonance (FMR) type of precession, a DMI-perturbed droplet forms and now remains stable for as long as the current density is limited to J =7.2 × 10 8 A cm −2 . When the current density is increased to J =8.3 × 10 8 A cm −2 the spin transfer torque provides enough energy to induce strong topological fluctuations between negative and positive skyrmion numbers to finally switch the system into a stable DS state. Once the DS has formed, the current density can be reduced substantially while still sustaining the precession, until a minimum sustaining current density is reached below which the DS rapidly collapses into a uniform ferromagnetic state, in a similar fashion as ordinary droplets. As a consequence it is perfectly possible to repeatedly access the uniform, droplet and DS states by only controlling the current density. By controlling both the drive current density and the applied field, transitions between all four states, including the static skyrmion, can be controlled at will, with the only limitation being the direct transformation of a skyrmion or DS into a droplet, which requires an intermediate step of a uniformly magnetized state. See Supplementary Movies 2 and 3 for the entire process of nucleation, field and current toggling of a DS in presence of DMI. Figure 6: Nucleation and current toggling of a DS in presence of DMI. Panels ( a – c ) show a DS nucleation as a function of current and fixed field, where the white circle indicates the NC of 15 nm radius. For 0 ns< t <1 ns, a magnetic droplet is nucleated when J =7.2 × 10 8 A cm −2 . For 1 ns< t <2 ns, a DS forms when current density is increased to 8.3 × 10 8 A cm −2 . For 2 ns< t <3 ns, a DS remains stable even when the current density is decreased to 6.7 × 10 8 A cm −2 , well below the threshold nucleation current density. For 3 ns< t <4 ns, the DS collapses into a uniform ferromagnetic state when the current density is further decreased to 6.3 × 10 8 A cm −2 . The current density is varied as follows: J =7.2 × 10 8 A cm −2 for 0< t <1 ns, 8.3 × 10 8 A cm −2 for 1 ns< t <2 ns, 6.7 × 10 8 A cm −2 for 2 ns< t <3 ns, and 6.3 × 10 8 A cm −2 for 3 ns< t <4 ns. Panel ( d ) schematically shows the current pulses applied during the simulation. Full size image In Fig. 7a,b we compare the field- and current-dependent tunability of the DS and the corresponding droplet (the latter simulated by removing the DMI term but otherwise sharing identical conditions). The most salient feature of the DS is a much stronger frequency tunability than the droplet. Whereas the droplet frequency is essentially independent of current density and linearly dependent on the field, the frequency of the DS decreases rapidly and linearly with increasing current density and exhibits a non-linear field dependence, in particular at low fields. In addition, the DS maximum frequency is bounded by its droplet counterpart. 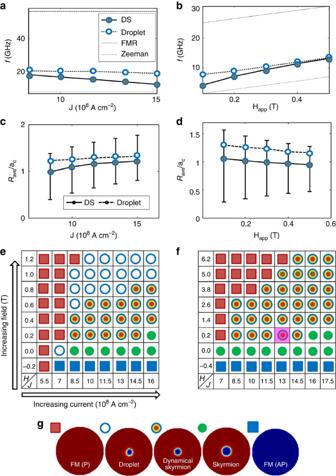Figure 7: Frequency, size and stability of DS. The frequency of the DS is shown as solid lines and filled circles for: (a)μ0Ha=0.3 T while the current density is varied; (b)J=8.3 × 108A cm−2while the applied field is varied. The corresponding droplet frequency (DMI=0) is shown as dotted lines and hollow circles. The Zeeman and FMR frequencies are shown as dashed lines. The radius of the droplet (hollow circles) and the time averaged radius of the DS (filled circles) measured in units of NC radius where the error bars indicate the total range of radii values as a function of: (c) current density; (d) applied perpendicular magnetic field strength. The DS frequency decreases rapidly with increasing radius (increasing current) ina. As the field increases inb, the DS becomes stiffer, reducing the breathing and making the dynamics resemble that of the droplet. (e) Nucleation of a droplet (hollow circle), DS (filled rainbow circle) and static skyrmion (green filled circle) at different fields and currents. (f) Sustainability of the DS over a very wide range of current and field. Note that the field axis is non-linear to reach the final collapse of the DS at very high fields. The DS was nucleated using the conditions highlighted by the pink square. (g) The schematic representation of different states. A droplet is represented by hollow circle; a DS is represented by filled rainbow circle; a static skyrmion is represented by green filled circle. The red and blue squares represent the upward and downward orientations of all the spins, respectively. Figure 7: Frequency, size and stability of DS. The frequency of the DS is shown as solid lines and filled circles for: ( a ) μ 0 H a =0.3 T while the current density is varied; ( b ) J =8.3 × 10 8 A cm −2 while the applied field is varied. The corresponding droplet frequency (DMI=0) is shown as dotted lines and hollow circles. The Zeeman and FMR frequencies are shown as dashed lines. The radius of the droplet (hollow circles) and the time averaged radius of the DS (filled circles) measured in units of NC radius where the error bars indicate the total range of radii values as a function of: ( c ) current density; ( d ) applied perpendicular magnetic field strength. The DS frequency decreases rapidly with increasing radius (increasing current) in a . As the field increases in b , the DS becomes stiffer, reducing the breathing and making the dynamics resemble that of the droplet. ( e ) Nucleation of a droplet (hollow circle), DS (filled rainbow circle) and static skyrmion (green filled circle) at different fields and currents. ( f ) Sustainability of the DS over a very wide range of current and field. Note that the field axis is non-linear to reach the final collapse of the DS at very high fields. The DS was nucleated using the conditions highlighted by the pink square. ( g ) The schematic representation of different states. A droplet is represented by hollow circle; a DS is represented by filled rainbow circle; a static skyrmion is represented by green filled circle. The red and blue squares represent the upward and downward orientations of all the spins, respectively. Full size image The key to understanding the much stronger field and current dependencies lies in the very strong breathing of the DS, which dominates the dynamics at large DMI. While the ordinary droplet is always slightly larger than the NC, and does not vary in size significantly with either current or field, the radius of the DS can at low fields have a minimum that is less than a third of the NC radius and a maximum that is more than 50% greater than the NC, as shown by the error bars in Fig. 7c,d . In other words, the breathing can make the DS radius vary by more than five times of its minimum size. The very strong breathing will increase the dissipation and the periodic motion of the domain-wall making up the DS perimeter will slow down the overall precession. When the current density is increased in Fig. 7c the maximum radius also increases, further slowing down the precession. However, when the field is increased in Fig. 7d the DS stiffens, the amplitude of the breathing decreases, and as a consequence, both the the maximum radius and the frequency of the DS approach those of the droplet. While in Fig. 7 we show the variation and average of the DS radius with the current, the change of the radius of the static skyrmion as a function of current is shown in Supplementary Fig. 9 . As observed in Fig. 6 above, the DS exhibits a similar degree of hysteresis as the original droplet, that is, its sustaining current can be much lower than the current needed for nucleation. This hysteresis ensures a minimum degree of stability, which should make the DS sufficiently robust for applications. In Fig. 7 , we investigate this stability in more detail and present a nucleation phase diagram in Fig. 7e and a stability phase diagram in Fig. 7f . The nucleation phase diagram presents the final steady state of the simulated system, when both current and field are turned on at t 0 and held constant until steady state. Five different end states can be identified as shown in Fig. 7g : a droplet, a DS, a static skyrmion, and the two saturated FM states. The stability phase diagram, on the other hand, presents the final steady state at all field and current values after a DS has first been nucleated at the conditions shown in pink. Here, only four different end states are possible as the DS never transforms back directly into a droplet. It is noteworthy that the DS is stable over a very large current and field range, more so than the droplet, which is consistent with its topological protection affording it additional stability. The DS is a solitonic, dynamical and topologically non-trivial magnetic structure which can be excited in NC-spin torque oscillators. A natural first application is therefore as a NC-spin torque oscillator based microwave signal generator where the DS has the potential to outperform both the original propagating [37] , [38] , [39] , [40] and localized [38] , [39] , [41] , [42] spin wave modes, as well as the recently discovered droplet [22] in a number of ways, including output power, minimum operating current density, current tunability, maximum operating frequency and microwave current injection locking. One of the most attractive properties of the original magnetic droplet soliton [21] , [23] , [24] is its much higher output power compared with the ordinary FMR-like precession, with experiments demonstrating a 40 × increase in output power as the droplet forms [22] . This is a consequence of the much larger precession angle, where a substantial fraction of the spins precess along the equator and hence make use (locally) of all the available magnetoresistance. While the DS also exhibits similarly large precession angles, its topological protection comes with a 2 π rotation of the relative phase along its perimeter, and as a consequence, the large in-plane precession averages out to zero microwave output power at all times. However, the very large breathing of the DS in materials exhibiting interfacial DMI restores the microwave signal. As the DS expands and contracts, m z of the local spins effectively varies between −1 and 1 at the same precessional frequency, as demonstrated theoretically above. Since the breathing can be >5 times the minimum DS diameter, which in turn is much smaller than the NC diameter, this mode essentially makes use of all the available perpendicular magnetoresistance of the device. As a consequence, the DS is expected to provide yet another order of magnitude increase in output power compared with the droplet, since in the latter, only the spins along the perimeter contribute their maximum power. As demonstrated experimentally in ref. 22 , the threshold current density for droplet nucleation in an orthogonal spin valve scales inversely with the applied out-of-plane field; the droplet nucleation is aided and the droplet is stabilized by the perpendicular component of the spin-polarized current density. The lowest threshold current density is consequently realized for a fixed layer that is saturated out-of-plane. However, since the droplet generates its microwave signal entirely from the in-plane component of its precession, it requires a significant in-plane component of the fixed layer magnetization for signal generation; a fully saturated fixed layer does not generate any microwave signal. Since the DS on the other hand derives its microwave signal entirely from the perpendicular magnetoresistance, it delivers its maximum output power exactly in the saturated fixed layer state. A DS-based NC-spin torque oscillator can hence simultaneously optimize for maximum output power and minimum operating current. A drawback of droplet based NC-spin torque oscillators is their poor current tunability, which limits both their frequency range and current modulation properties. However, as shown in Fig. 7c above, the breathing of the DS provides for a very large current tunability, which makes it much more attractive for broadband microwave applications. As shown in Fig. 7f above, the DS is inherently stable even at very high fields. Consequently, it can operate at a much higher frequency than the droplet, which is limited by the saturation field of its fixed layer. While the droplet is essentially insensitive to injection locking to a microwave current ( Fig. 8a ), the DS is readily injection locked ( Fig. 8b ), primarily due to strong coupling between the time-varying spin transfer torque and the breathing. This sensitivity is not only important in microwave sensor applications, it also provides direct means to mutually synchronize a large number of DS-based NC-spin torque oscillators in series via their shared microwave current [43] , [44] , [45] , [46] . The dramatic difference in injection locking strength and the strong current dependence of the frequency are likely the most straightforward experimental tests for a first experimental demonstration of a DS. The DS also holds great potential for direct skyrmionic applications driven by the rich interactions between droplets, DSs and static skyrmions. To illustrate, we here provide one intriguing example of a droplet based ultrafast read-out of a skyrmion. As our intial condition we take a static skyrmion in proximity to a NC ( Fig. 9 ). We then pass enough current through the NC to nucleate a droplet without driving a transition to a DS. As the DMI driven perturbations of the droplet rotate around the NC, they interact with the nearby skyrmion, which eventually feels enough of an attractive force to be pulled in underneath the NC where it merges with the droplet and in the process transfers its topology, transforming the droplet into a DS (see Supplementary Movie 4 ). This transformation can be observed in the time-frequency representation of Fig. 9d (see the Methods section) where, within a fraction of a nanosecond, the spins change their precession frequency from ∼ 30 to 20 GHz and the characteristic breathing starts, instantly generating a microwave signal across the device. 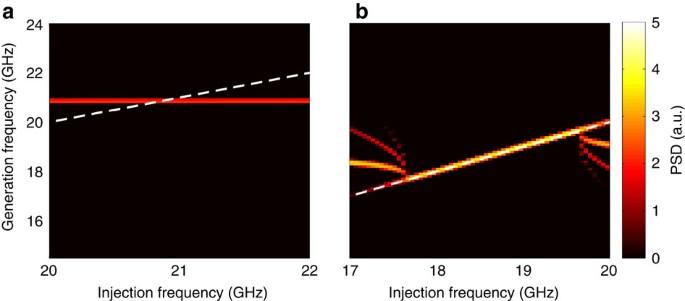Figure 8: Droplet and DS injection locking. Injection locking diagram of (a) a droplet and (b) a DS as a function of the frequency of the injected microwave current (white dashed lines). The injected signal is a pure tone with amplitude 0.2 times the bias current density. The full current-induced Oe field is also included in these simulations. While the droplet is not visibly injection locked for the considered parameters, the DS exhibits a very large phase locking bandwidth of∼3 GHz. Outside of the locked region the DS exhibits strong intermodulation products further demonstrating its strong interaction with the injected current. Figure 8: Droplet and DS injection locking. Injection locking diagram of ( a ) a droplet and ( b ) a DS as a function of the frequency of the injected microwave current (white dashed lines). The injected signal is a pure tone with amplitude 0.2 times the bias current density. The full current-induced Oe field is also included in these simulations. While the droplet is not visibly injection locked for the considered parameters, the DS exhibits a very large phase locking bandwidth of ∼ 3 GHz. Outside of the locked region the DS exhibits strong intermodulation products further demonstrating its strong interaction with the injected current. 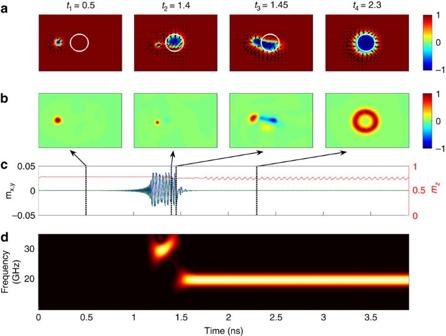Figure 9: Droplet nucleation and skyrmion read-out. (a) and (b) are the top views of the spin structure and normalized topological density at four different times; (c) time trace of the three magnetisation components averaged over the simulation area with dashed vertical lines corresponding to the snapshots above; (d) time-dependent frequency of the precessing magnetization. A static skyrmion is initialized as the micromagnetic ground state att1. By applying a current densityJ=7.2 × 108A cm−2, a droplet is nucleated (t2). The droplet acts as an attractive source for the static skyrmion until it merges att3. The droplet absorbs the skyrmion topology as evidenced by the reduction of the in-plane magnetisation and the frequency drop as the DS forms at (t4). Full size image Figure 9: Droplet nucleation and skyrmion read-out. ( a ) and ( b ) are the top views of the spin structure and normalized topological density at four different times; ( c ) time trace of the three magnetisation components averaged over the simulation area with dashed vertical lines corresponding to the snapshots above; ( d ) time-dependent frequency of the precessing magnetization. A static skyrmion is initialized as the micromagnetic ground state at t 1 . By applying a current density J =7.2 × 10 8 A cm −2 , a droplet is nucleated ( t 2 ). The droplet acts as an attractive source for the static skyrmion until it merges at t 3 . The droplet absorbs the skyrmion topology as evidenced by the reduction of the in-plane magnetisation and the frequency drop as the DS forms at ( t 4 ). Full size image In summary, we have shown the existence of a dynamically stabilized skyrmion which may exist in a large range of material parameters including materials where DMI is entirely absent. Carrying the hallmark of a quasiparticle, the DS can be reversibly transported between NCs in the presence of dissipation. In the presence of DMI, the DS exhibits strong breathing and thus has great potential for both new physics and direct applications in skyrmionics and NC-based microwave signal generators. Micromagnetic simulations Micromagnetic simulations are performed for the free layer with the graphics-processing-unit-based tool Mumax3 (ref. 30 ). The time-dependent spin dynamics follow the Landau–Lifshitz–Gilbert–Slonczewski equation of motion, where | γ |/2 π =28 GHz T −1 is the gyromagnetic ratio, α is the Gilbert damping parameter, μ 0 is the magnetic vacuum permeability, M s is the free-layer saturation magnetisation and m is the free-layer magnetisation unit vector. The fixed layer magnetisation vector is along . is the spin torque coefficient where ℏ is the reduced Planck constant, I is the electric current, P is spin polarization, e is the elementary charge ( e >0), V is the volume of the magnetization within the NC range. , where λ is the magnetoresistance asymmetry parameter describing the deviation from sinusoidal angular dependence. is the Heaviside step function approximately describing the current distribution, that is, for and 0 otherwise. The effective field includes the contribution from Heisenberg exchange, perpendicular magnetic anisotropy, DMI, and an applied external field along the direction. The DMI in Mumax3 is assumed to be purely of interfacial origin, giving rise to the contribution to the energy density [47] . where D is the DMI constant. A NC-spin torque oscillator geometry is modelled, based on a pseudo spin valve with perpendicular magnetic anisotropy fixed and free layers and a current-confining NC of radius 15 nm placed at the centre of the free layer (except in Fig. 2 and Fig. 3 where the NC radius is chosen to be either 30 or 40 nm). The free layer is assumed to be a 1 nm thick Co film with radius of 100 nm on a substrate inducing DMI, which can be controlled by varying the layer thickness, and material parameters similar to ref. 14 , namely: exchange constant A =15 pJ m −1 , Gilbert damping α =0.3, spin polarization ratio P =0.3, saturation magnetisation M s =580 kA m −1 , D =3 mJ m −2 and K u =0.7 MJ m −3 unless otherwise specified. Note that the assumed strength of the DMI corresponds to values reported in Pt/Co/AlO x thin films [48] , where πD 0 ∼ 0.7. These parameters lead to a domain-wall width of δ 0 =4.6 nm. The fixed layer is assumed to be magnetised along the +z direction, inducing a spin transfer torque with λ =1 for simplicity. All of our simulations are performed with unit cell size between 1 and 2 nm, which is well below δ 0 and the exchange length, ensuring numerical accuracy. For finite temperature simulations in Supplementary Note 4 , a fixed time step of 0.1 fs is used. The simulations are performed with open boundary conditions, that is, damping is set to be uniform across the whole disk including the boundary (for details see Supplementary Note 4 and Supplementary Figs 10–13 ). Time-frequency diagram The time-frequency diagram of Fig. 9d is obtained by performing the smoothed pseudo Wigner–Ville transform. This transform is superior than the well-known spectrograms or scalograms as it offers arbitrary resolution in time and frequency at the expense of computational artifacts. Such artifacts are greatly removed by performing time and frequency smoothing. Here a Gaussian function is used to smooth time while a Hann window is used to prevent spectral leakage. In the particular case of Fig. 9d , we use a 0.2 ns wide Gauss function and a 3 GHz Hann window. How to cite this article: Zhou, Y. et al. Dynamically stabilized magnetic skyrmions. Nat. Commun. 6:8193 doi: 10.1038/ncomms9193 (2015).